Coordination tailoring of Cu single sites on C3N4realizes selective CO2hydrogenation at low temperature CO 2 hydrogenation has attracted great attention, yet the quest for highly-efficient catalysts is driven by the current disadvantages of poor activity, low selectivity, and ambiguous structure-performance relationship. We demonstrate here that C 3 N 4 -supported Cu single atom catalysts with tailored coordination structures, namely, Cu–N 4 and Cu–N 3 , can serve as highly selective and active catalysts for CO 2 hydrogenation at low temperature. The modulation of the coordination structure of Cu single atom is readily realized by simply altering the treatment parameters. Further investigations reveal that Cu–N 4 favors CO 2 hydrogenation to form CH 3 OH via the formate pathway, while Cu–N 3 tends to catalyze CO 2 hydrogenation to produce CO via the reverse water-gas-shift (RWGS) pathway. Significantly, the CH 3 OH productivity and selectivity reach 4.2 mmol g –1 h –1 and 95.5%, respectively, for Cu–N 4 single atom catalyst. We anticipate this work will promote the fundamental researches on the structure-performance relationship of catalysts. CO 2 hydrogenation has attracted great attention because it can simultaneously reduce the CO 2 emission [1] , [2] , [3] , [4] and produce high value-added chemicals [5] , [6] , [7] , [8] , yet it suffers from low activity and selectivity due to the chemical inertness of CO 2 and the complicated process of CO 2 hydrogenation [9] , [10] , [11] . To promote CO 2 hydrogenation, one needs to raise the temperature or pressure, which however results in increased selectivity of CO and decreased selectivities of value-added chemicals. For instance, Cu-based catalysts have been widely used for CO 2 hydrogenation, which are generally operated at temperature and pressure ranges of 220–300 °C and 50–100 atm, respectively [10] , [11] . Over the past decades, great efforts have been devoted to developing efficient catalysts for CO 2 hydrogenation, such as compositing Cu sites with metal oxides (e.g., ZnO, ZrO 2 , and TiO 2 ) [12] , [13] , [14] , [15] , [16] , [17] , [18] , [19] , [20] . However, the request for efficient CO 2 hydrogenation catalysts is driven by the current drawbacks including poor activity and/or CH 3 OH selectivity, as well as the ambiguous mechanism. Recently, single atom catalysts (SACs) have attracted great attention in catalysis due to their properties including 100% atom utilization efficiency, low coordination environment, confinement effect, etc [21] , [22] , [23] , [24] , [25] , [26] , [27] , [28] , [29] , [30] . Typical for CO 2 hydrogenation, SACs are regarded as promising catalysts for producing high value-added chemicals. For instance, Ye et al. synthesized Ir 1 –In 2 O 3 SAC for CO 2 hydrogenation with a high C 2 H 5 OH selectivity of 99% and a turnover frequency (TOF) value of 481 h –1 [31] . It is found that CO 2 can be activated into CO * on the isolated Ir atom, and then couples with the methoxide adsorbed on the In 2 O 3 to form C–C bond. Zhang and co-workers fabricated a stable Ir-based SAC for CO 2 hydrogenation to formate. Detailed characterizations and theoretical calculations indicate that such Ir-based SAC has a similar structure with a homogeneous mononuclear Ir pincer complex catalyst, which can serve as an efficient catalyst for the conversion of CO 2 to formate [32] . Despite this progress, CO 2 hydrogenation to value-added liquid products over SACs is still far away from the satisfaction of chemical industry because of the following issues: (1) it is challenging to precisely regulate the selectivities of products during CO 2 hydrogenation over SACs, (2) the poor stability of SACs at high temperature and pressure needs to be overcome, and (3) the intrinsic structure-performance relationship of SACs has not been clearly understood yet. It is thus highly desired to develop efficient SACs with enhanced activity, selectivity and stability for CO 2 hydrogenation under mild conditions. In this work, we used C 3 N 4 , a functional support with abundant N sites, to anchor Cu single sites for CO 2 hydrogenation at a low temperature range of 70–150 °C. By simply altering the treatment conditions, the coordination structures of Cu single atoms can be regulated, for instance, Cu–N 4 and Cu–N 3 structures. Experimental results imply that Cu–N 3 SAC displays a CO selectivity of 94.3%, while Cu–N 4 SAC exhibit a CH 3 OH selectivity of 95.5% at a CH 3 OH productivity of 4.2 mmol g –1 h –1 at 150 °C. Impressively, the CH 3 OH productivity for Cu–N 4 SAC has surpassed the state-of-the-art Cu-ZnO/Al 2 O 3 by 3.2 times (1 mmol g –1 h –1 ). Moreover, Cu–N 4 SAC shows promising stability without decay of CH 3 OH productivity and changes in the structure after 5 consecutive cycles. Further studies imply that CO 2 hydrogenation follows the formate pathway to form CH 3 OH on Cu–N 4 SAC and the RWGS pathway to form CO on Cu–N 3 SAC, respectively. This work not only provides an efficient SAC for CO 2 hydrogenation to form CH 3 OH under mild conditions, but also sheds interesting light on studying the structure-performance relationship of catalyst. Structure analysis of catalysts C 3 N 4 supported Cu SACs were synthesized via the thermal pyrolysis of melamine (see experimental section for details). 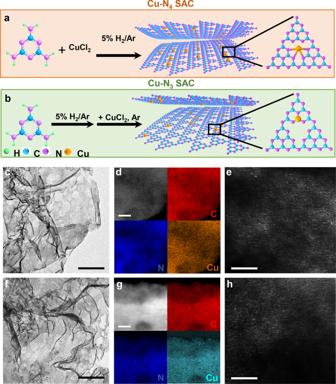Fig. 1: Scheme for the synthesis and characterizations of Cu–N4and Cu–N3SACs. Scheme for the synthesis of (a) Cu–N4and (b) Cu–N3SACs.cTEM image, (d) element mapping images, and (e) magnified HAADF-STEM image of Cu–N4SAC.fTEM image, (g) element mapping images, and (h) magnified HAADF-STEM image of Cu–N3SAC. The scale bars in (c–h) are 200, 20, 2, 200, 20, and 2 nm, respectively. The physicochemical properties of catalysts including the compositions (determined by inductively coupled plasma-atomic emission spectroscopy (ICP-AES) measurement) are listed in Supplementary Table 1 . Results from the N 2 adsorption–desorption measurement suggest the generation of mesopores in Cu–N 4 and Cu–N 3 SACs. Consequently, the surface areas of pristine C 3 N 4 , Cu–N 4 SAC and Cu–N 3 SAC are 0.70, 22.5, and 20.8 m 2 /g, respectively (Supplementary Fig. 1 ). Transmission electron microscopy (TEM) image shows that the as-prepared C 3 N 4 displays a morphology of nanosheet (Supplementary Fig. 2 ). C 3 N 4 supported Cu SACs with tailored coordination environment, namely, Cu–N 4 and Cu–N 3 SACs, were generated by depositing CuCl 2 onto C 3 N 4 under specific conditions (Fig. 1a, b ). After loading Cu on C 3 N 4 , no obvious changes in the morphologies of Cu–N 4 and Cu–N 3 SACs are observed (Fig. 1c, f ). Scanning transmission electron microscopy energy-dispersive X-ray spectroscopy (STEM-EDS) images indicate that Cu, C, and N are well dispersed in the Cu–N 4 and Cu–N 3 SACs (Fig. 1d, g ). Moreover, the atomic ratios of Cu in Cu–N 4 and Cu–N 3 SACs are 12.1% and 13.1%, respectively (Supplementary Fig. 3 ), which are close to those values from ICP-AES measurement (Supplementary Table 1 ). Atomic force microscopy (AFM) images demonstrate that Cu–N 4 and Cu–N 3 SACs have similar thicknesses with C 3 N 4 (~1.6 nm, Supplementary Fig. 4 ). Note that the decrease of thickness of Cu–N 4 and Cu–N 3 SACs compared with the pristine C 3 N 4 might be attributed to the delamination of C 3 N 4 during the synthesis of SACs. Moreover, spherical aberration TEM (SA-TEM) measurement was employed to study the states of Cu atoms in different samples. It is found that Cu atoms, which are presented as dense white dots, display as single state in the Cu–N 4 and Cu–N 3 SACs (Fig. 1e, h ). On the other hand, Cu NPs with a mean size of 3 nm are observed in the C 3 N 4 supported Cu nanoparticles (Cu NPs/C 3 N 4 ) (Supplementary Fig. 2b ). The structures of Cu–N 4 and Cu–N 3 SACs were studied by X-ray diffraction (XRD) measurement. In the XRD pattern of C 3 N 4 , typical peaks appear at 2θ of 13.1° and 27.3°, which are ascribed to (100) and (002) facet, respectively (black curve in Supplementary Fig. 5 ). No obvious differences in the XRD patterns of Cu–N 4 and Cu–N 3 SACs are attributed to the isolated state of Cu atom (red and blue curves in Supplementary Fig. 5 ). By contrast, the typical peaks of Cu NPs appear at 43.3°, 50.4°, and 74.1° in the XRD pattern of Cu NPs/C 3 N 4 , which correspond to the characteristic peaks of Cu (111), (200), and (220) facets, respectively (Supplementary Fig. 6 ). Moreover, the peaks at 3145, 1639, 1145, and 798 cm –1 in the Fourier transform infrared spectroscopy (FTIR) spectrum of C 3 N 4 can be indexed as the stretching vibrations of triazine ring, –NH 2 , –OH, and the bending vibration of triazine ring, respectively, and the presence of characteristic peaks of C 3 N 4 in the FTIR spectra of Cu–N 4 and Cu–N 3 SACs suggested that the structure of C 3 N 4 is largely maintained after Cu loading (Supplementary Fig. 7 ). Fig. 1: Scheme for the synthesis and characterizations of Cu–N 4 and Cu–N 3 SACs. Scheme for the synthesis of ( a ) Cu–N 4 and ( b ) Cu–N 3 SACs. c TEM image, ( d ) element mapping images, and ( e ) magnified HAADF-STEM image of Cu–N 4 SAC. f TEM image, ( g ) element mapping images, and ( h ) magnified HAADF-STEM image of Cu–N 3 SAC. The scale bars in ( c – h ) are 200, 20, 2, 200, 20, and 2 nm, respectively. Full size image X-ray photoelectron spectroscopy (XPS) measurement was further used to reveal the surface properties of SACs. It is found that the surface of Cu NPs is partially oxidized, as presented by the shoulders at 934.7 and 955.0 eV in the XPS spectrum of Cu NPs/C 3 N 4 (Fig. 2a ). Considering the appearance of Cu peaks in the XRD pattern of Cu NPs/C 3 N 4 (Supplementary Fig. 6 ), the peaks at 932.5 and 952.2 eV are ascribed to 2 p 1/2 and 2 p 3/2 peaks of Cu 0 . For Cu–N 4 SACs, the characteristic peaks of Cu + 2 p 2/3 and 2 p 1/2 appear at 932.5 and 952.2 eV, respectively (Note that the peaks of Cu 0 and Cu + locates at similar positions in XPS spectrum). For Cu–N 3 SACs, in addition to the features of Cu + , two peaks corresponding to Cu 2+ appear at 935.0 and 955.0 eV in the Cu 2 p XPS spectrum with a Cu 2+ /Cu + ratio of ~2 (Fig. 2a ). For N 1 s XPS spectra of Cu–N 4 and Cu–N 3 SACs, the features of pyridinic N, pyrrolic-N and graphic-N are observed at 398.6, 400.2 and 401.3 eV, respectively, which are similar to those of C 3 N 4 (Supplementary Fig. 8 ). Moreover, the oxidation states of Cu in Cu–N 4 and Cu–N 3 SACs have been further confirmed by Auger Electron Spectroscopy (AES) spectra, in which the peaks negatively shift to lower binding energies compared with Cu NPs/C 3 N 4 (Supplementary Fig. 9 ). To further reveal the chemical states of Cu atoms in Cu–N 4 and Cu–N 3 SACs, diffuse reflectance infrared Fourier transform spectroscopy (DRIFTS) measurement using CO as the probe molecule was performed. Two weak bands appear at 2173 and 2119 cm –1 in the CO-DRIFTS spectra of Cu–N 4 and Cu–N 3 SACs, which are ascribed to CO linear adsorption on Cu atoms (Fig. 2b ). Additionally, X-ray absorption near-edge structure (XANES) and extended X-ray absorption fine structure (EXAFS) measurement were performed at Cu K-edge to investigate the local structures of Cu atoms in catalysts. Compared to Cu foil, the absorption edges for Cu–N 4 and Cu–N 3 SACs shift to higher energy, suggesting the oxidation states of Cu in Cu–N 4 and Cu–N 3 SACs (Fig. 2c ). Moreover, we estimated the mean chemical valences of Cu in Cu–N 4 and Cu–N 3 SACs based on the XANES spectra of Cu–N 4 SAC, Cu–N 3 SAC, Cu foil, Cu 2 O, and CuO. As shown in Supplementary Fig. 10 , the mean chemical valences of Cu in Cu–N 4 and Cu–N 3 SACs are +1.05 and +1.64, respectively. In the EXAFS spectra of Cu 2 O and CuO, the peaks at 1.55 and 2.23 Å are ascribed to the coordination of Cu–O and Cu–Cu, respectively (Fig. 2d ). The absences of Cu–Cu coordination in the EXAFS spectra of Cu–N 4 and Cu–N 3 SACs suggest that Cu atoms are presented as isolated state (Fig. 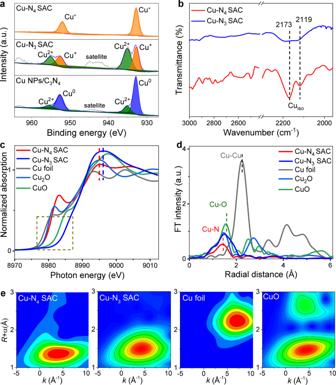Fig. 2: Structural characterizations of various catalysts. aXPS spectra of Cu–N4SAC, Cu–N3SAC, and Cu NPs/C3N4.bCO-DRIFT spectra of Cu–N4and Cu–N3SACs.cXANES and (d) EXAFS spectra of Cu–N4SAC, Cu–N3SAC, Cu foil, Cu2O, and CuO at CuK-edge.eWavelet transform of EXAFS spectra at CuK-edge. Source data are provided as aSource Data file. 2d and Supplementary Table 2 ). Additionally, wavelet transform (WT) at the Cu K-edge EXAFS analysis further confirms the isolated state of Cu atoms in Cu–N 4 and Cu–N 3 SACs. As shown in Fig. 2e , the intense Cu–N coordination, which is illustrated by red color, is observed in the WT contour plots of Cu–N 4 SAC and Cu–N 3 SAC at the radial distances of ~1.45 Å (Y axis). Also, the strong Cu–Cu (~2.2 Å) and Cu–O (1.5 Å) coordination can be observed in the WT contour plots of Cu foil and CuO, which agrees with the results from EXAFS spectra (Fig. 2e ). Fig. 2: Structural characterizations of various catalysts. a XPS spectra of Cu–N 4 SAC, Cu–N 3 SAC, and Cu NPs/C 3 N 4 . b CO-DRIFT spectra of Cu–N 4 and Cu–N 3 SACs. c XANES and ( d ) EXAFS spectra of Cu–N 4 SAC, Cu–N 3 SAC, Cu foil, Cu 2 O, and CuO at Cu K -edge. e Wavelet transform of EXAFS spectra at Cu K -edge. Source data are provided as a Source Data file . Full size image CO 2 hydrogenation The performance of CO 2 hydrogenation was evaluated in a batch stainless-steel reactor with 10 mg catalyst and 10 mL water. Commercial Cu-ZnO/Al 2 O 3 , C 3 N 4 , and Cu NPs/C 3 N 4 were used as references. Prior to catalytic tests, the reactor was pre-flushed with N 2 for five times. Afterwards, a mixture of H 2 , CO 2 , and N 2 (72:24:4 vol.%) was pressurized into the reactor with a total pressure of 3.2 MPa. As shown in Fig. 3a , no gaseous (e.g., CO and CH 4 ) and liquid products (e.g., CH 3 OH) were detected at 150 °C when C 3 N 4 was as catalyst, indicating that C 3 N 4 is inactive under the indicated conditions. When Cu NPs/C 3 N 4 was used as catalyst, CH 3 OH productivity is 1.8 mmol g –1 h –1 at a CH 3 OH selectivity of 78.6%. CH 3 OH productivity significantly increases to 4.2 mmol g –1 h –1 at a CH 3 OH selectivity of 95.5% for Cu–N 4 SAC. In contrast, CO selectivity reaches 94.3% with a CO productivity of 2.5 mmol g –1 h –1 when Cu–N 3 SAC was used as catalyst. It is noted that the productivity and selectivity of CH 3 OH for Cu–N 4 SAC are much higher than those of Cu NPs/C 3 N 4 (Supplementary Fig. 11 ) and commercial Cu-ZnO/Al 2 O 3 (Supplementary Fig. 12 ). Moreover, CH 3 OH and CO productivities reach 4.2 and 2.5 mmol g –1 h –1 , respectively, when the reaction time was extended to 3 h. As shown in Fig. 3c , when Cu–N 4 SAC was used as catalyst, the CH 3 OH productivity increases from 0.6 to 4.2 mmol g –1 h –1 with the increased temperature from 70 to 150 °C, whereas the selectivity of CH 3 OH is kept at ~95%. On the other hand, the CO productivity increases from 0.2 to 2.6 mmol g –1 h –1 for Cu–N 3 SAC when the reaction temperature was elevated from 70 to 150 °C (Fig. 3c ). We also evaluated the catalytic performance at the temperature range from 70 to 150 °C (Supplementary Figs. 13 , 14 ). It is found high temperature favors CO 2 hydrogenation over Cu–N 4 (to produce CH 3 OH) and Cu–N 3 (to produce CO) SACs. The above results indicate that Cu–N 4 SAC can serve as highly active and selective catalyst for CO 2 hydrogenation to CH 3 OH, while Cu–N 4 SAC favors for CO formation (Fig. 3b ). Moreover, the kinetics for CO 2 hydrogenation were studied for further evaluating the catalytic performance. Arrhenius plots indicate that the apparent activation energies (Ea) for the commercial Cu-ZnO/Al 2 O 3 , Cu NPs/C 3 N 4 , Cu–N 4 SAC, and Cu–N 3 SAC are 130.6, 130.3, 50.2, and 86.6 kJ mol –1 , respectively (Fig. 3d ). The smallest value of Ea for Cu–N 4 SAC indicates that Cu–N 4 SAC can serve as the most active catalyst for CO 2 hydrogenation, which is consistent with our experimental observations. We further calculated the reaction orders with respect to CO 2 and H 2 for Cu–N 4 SAC, and the reaction orders of CO 2 and H 2 are 1.18 and 1.19, respectively (Supplementary Fig. 15 ). 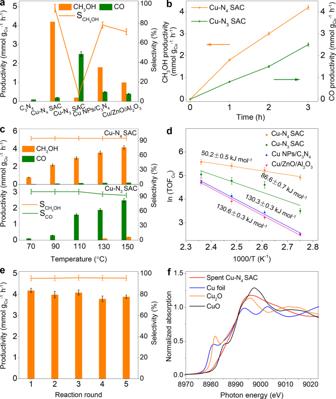Fig. 3: Catalytic performance of CO2hydrogenation. aCatalytic performance of CO2hydrogenation over different catalysts.bCH3OH and CO productivities of Cu–N3SAC and Cu–N4SAC, respectively. Reaction conditions for (a) and (b): H2/CO2/N2= 72:24:4 vol.%,Ptotal= 3.2 MPa,T= 150 °C, and reaction time is 3 h.cCO2hydrogenation over Cu–N4and Cu–N3SACs at different temperatures. Reaction conditions: H2/CO2/N2= 72:24:4 vol.%,Ptotal= 3.2 MPa,T= 70–150 °C, and reaction time is 3 h.dArrhenius plots of different catalysts.eCH3OH productivity and selectivity over Cu–N4SAC in 5 cycles. Reaction conditions: H2/CO2/N2= 72:24:4 vol.%,Ptotal= 3.2 MPa,T= 150 °C, and the reaction time for each cycle is 3 h.fXANES spectra of the spent Cu–N4SAC. All the data in (a–e) were collected for three times, and the error bars represent the standard deviation. Source data are provided as aSource Data file. Note that the catalytic performance of Cu–N 4 SAC has surpassed most of the reported Cu-based catalysts for CO 2 hydrogenation (Supplementary Table 3 ). Fig. 3: Catalytic performance of CO 2 hydrogenation. a Catalytic performance of CO 2 hydrogenation over different catalysts. b CH 3 OH and CO productivities of Cu–N 3 SAC and Cu–N 4 SAC, respectively. Reaction conditions for ( a ) and ( b ): H 2 /CO 2 /N 2 = 72:24:4 vol.%, P total = 3.2 MPa, T = 150 °C, and reaction time is 3 h. c CO 2 hydrogenation over Cu–N 4 and Cu–N 3 SACs at different temperatures. Reaction conditions: H 2 /CO 2 /N 2 = 72:24:4 vol.%, P total = 3.2 MPa, T = 70–150 °C, and reaction time is 3 h. d Arrhenius plots of different catalysts. e CH 3 OH productivity and selectivity over Cu–N 4 SAC in 5 cycles. Reaction conditions: H 2 /CO 2 /N 2 = 72:24:4 vol.%, P total = 3.2 MPa, T = 150 °C, and the reaction time for each cycle is 3 h. f XANES spectra of the spent Cu–N 4 SAC. All the data in ( a – e ) were collected for three times, and the error bars represent the standard deviation. Source data are provided as a Source Data file . Full size image Additionally, the stability of Cu–N 4 SAC was evaluated in five consecutive cycles at 150 °C. No obvious decay of the CH 3 OH productivity indicates the promising stability of Cu–N 4 SAC for CO 2 hydrogenation (Fig. 3e ). Besides, the local structures of Cu atoms are largely maintained for the spent Cu–N 4 SAC (Fig. 3f , Supplementary Figs. 16 , 17 ). ICP-AES results indicate that the content of Cu in spent Cu–N 4 SAC is close to that of fresh Cu–N 4 SAC (10.2%), confirming the enhanced stability of Cu–N 4 SACs for CO 2 hydrogenation. Additionally, in situ IR (Supplementary Fig. 18 ) and XRD measurements were performed for Cu–N 4 and Cu–N 3 SACs for further studying the stability of Cu–N 4 SAC for CO 2 hydrogenation. No obvious changes are observed in the IR spectra collected at 3 MPa and 150 °C with different reaction times, suggesting the promising stabilities of catalysts for CO 2 hydrogenation (Supplementary Fig. 19 ). In particular, the peak at 3170, 1650, 1175 and 808 cm -1 are ascribed to the vibrations of triazine ring stretching, –NH 2 , –OH stretching, and triazine ring bending, respectively. Besides, in situ XRD patterns were collected at different temperature and in the presence of H 2 /CO 2 /N 2 (72:24:4 vol.%) with a total pressure of 0.03 MPa. As shown in Supplementary Fig. 20 , the peak at 27.3° can be indexed as the (002) facet of C 3 N 4 , and no obvious changes were observed when the temperature was increased from 40 to 150 °C, further confirming the enhanced stability of Cu–N 4 SAC. Note that the slight decrease of productivity in 5 cycles might be attributed to the catalyst loss during centrifugation. Catalysis mechanism studies To understand the distinct performance and catalysis mechanism of Cu–N 4 and Cu–N 3 SACs towards CO 2 hydrogenation, in situ DRIFTS measurement was performed by exposing different catalysts to a mixture of CO 2 and H 2 (1:3 vol.%) at 0.1 MPa and 150 °C. No peaks were observed in the DRIFTS spectra before introducing CO 2 and H 2 onto Cu–N 4 and Cu–N 3 SACs (red curves in Supplementary Fig. 21a, b ). After the introduction of CO 2 and H 2 , several peaks appear at 3265, 2964, 2848, 2514, 2014, and 1917 cm –1 in the DRIFTS spectrum of Cu–N 4 SAC, which can be indexed as the characteristic peaks of CH 3 O * (Supplementary Fig. 21a ). In contrast, two weak peaks are observed at 2114 and 2176 cm –1 in the DRIFTS spectrum of Cu–N 3 SAC, which are ascribed to CO * adsorption (Supplementary Fig. 21b ). Additionally, given the significant differences in the coordination environment of Cu–N 4 SAC (consists of Cu + ) and Cu–N 3 SAC (consists of Cu + and Cu 2+ ), we further studied the effects of Cu 2+ /Cu + ratio on the performance of CO 2 hydrogenation. Considering H 2 can reduce Cu 2+ into Cu + , we thus treated Cu–N 3 SAC at 500 °C for different times. In particular, the Cu 2+ /Cu + ratios are 1 and 0.5 when Cu–N 3 SAC was treated at 500 °C for 15 and 30 min, respectively. When the Cu 2+ /Cu + ratio is increased from 0.5 to 2 (Supplementary Fig. 22 ), CH 3 OH productivity significantly decreases from 2.8 to 0.25 mmol g –1 h –1 , while CO productivity significantly increases from 0.5 to 2.6 mmol g –1 h –1 (Supplementary Fig. 23 ). The aforementioned results imply that the catalytic performance of CO 2 hydrogenation was strongly depended on the coordination environment of Cu atoms. Density functional theory (DFT) calculations were further performed to confirm the stable configurations of Cu single atoms on C 3 N 4 and the corresponding mechanism for catalysis. We choose the buckled C 3 N 4 structure as the substrate, because it is more stable than the planar one, which has been fully discussed in the previous studies [33] , [34] , [35] . EXAFS analysis indicates that the coordination numbers of Cu–N for Cu–N 3 and Cu–N 4 SACs are ~3.1 and 3.7, respectively (Supplementary Table S2 ), we thus selected two models to mimic the structures of Cu single atoms on C 3 N 4 : 1) Cu atom locates at the hole site of C 3 N 4 (Supplementary Fig. 24 ). After structural relaxation, Cu atom will not locate at the center of the hole but slightly moves to one side. Cu atom strongly coordinates with two N atoms with the bond length of 2.18 Å and 2.16 Å, and two longer Cu–N bonds of 2.28 Å and 2.38 Å are also formed. In this model, Cu atom is coordinated with 4 N atoms to form structure of Cu–N 4 , which is consistent with the results from EXAFS measurement. The adsorption energy of Cu is 2.98 eV, which is higher than the adsorption energy of Pd single atoms on C 3 N 4 (2.17 eV) in previous work [36] , indicating that Cu atoms can be firmly anchored on C 3 N 4 in single state; 2) Cu atom replaces one of C atoms in C 3 N 4 to form three Cu–N bonds (Supplementary Fig. 25 ). In this model, Cu is coordinated with 3 N atoms, and the length of Cu–N bond is as short as ~1.80 Å, indicating a strong coordination between Cu and N atoms. To confirm the thermodynamic stability of our two models, we have performed the molecular dynamics (MD) calculations at the temperature of 450 K for totally 10 ps with a time step of 1 fs for both Cu–N 3 and Cu–N 4 , respectively. From our results, we can observe the fluctuation of the total energy with the time evolution, as shown in Supplementary Fig. 26 . The energies are oscillating near the equilibrium state and there is no structural disruption throughout simulations, indicating the two models are thermodynamically stable. Furthermore, we estimated the Bader charges of Cu in the above two models. It is found that the Bader charge of Cu in Cu–N 3 model is +0.95e, which is larger than that of Cu–N 4 model (+0.73e), suggesting that more electrons transfer from Cu to neighboring N atoms in Cu–N 3 model compared to Cu–N 4 model (Supplementary Fig. 27 ). Consequently, the valence of Cu in Cu–N 3 is higher than that in Cu–N 4 , which is consistent with the results from XANES measurement. Additionally, we analysed the projected density of states (PDOS) of Cu in Cu–N 3 and Cu–N 4 models to study the electronic structures. It is found that the 3d orbital of Cu atom strongly couples with the 2p orbital of N atom, which confirms the strong coordination between Cu single atoms and C 3 N 4 (Fig. 4a, b ). Compared to Cu–N 4 ( + 0.73e), the orbital coupling between Cu and N atoms for Cu–N 3 (+0.95e) shifts to lower energy levels (far away from the Fermi level), indicating a relatively higher valence state of Cu, which is in agreement with characterizations and Bader charge analysis. We finally simulated the K -edge XANES spectra of Cu–N 4 and Cu–N 3 SACs based on the selected models. As shown in Supplementary Fig. 28 , it is found that both the simulated XANES spectra of Cu–N 4 and Cu–N 3 models display similar features with those of the original ones, further indicating that the selected Cu–N 4 and Cu–N 3 models are representative for investigating the mechanism for catalysis. Fig. 4: Theoretical calculations and possible reaction paths for CO 2 hydrogenation. Projected density of states for ( a ) Cu–N 4 and ( c ) Cu–N 3 SACs, and the Fermi level is indicated by the dashed line. Energy profiles for ( b ) CO 2 hydrogenation via formate pathway over Cu–N 4 SAC and ( d ) CO 2 hydrogenation via RWGS pathway over Cu–N 3 SAC. Reaction pathways and corresponding atomic configurations for CO 2 hydrogenation to ( e ) CH 3 OH and ( f ) CO. The temperature is set as 423 K. The yellow, blue, gray, red and white balls in ( e ) and ( f ) represent as Cu, N, C, O, and H atoms, respectively. Full size image Moreover, DFT calculations were conducted to investigate the reaction pathways of CO 2 hydrogenation on Cu–N 4 and Cu–N 3 SACs. Based on the previous reports [19] , [20] , the major reaction pathway for CO formation is the reverse-water-gas-shift (RWGS) reaction via carboxyl ( * HOCO) intermediate, while the formation of CH 3 OH involves a formate pathway. We then systematically investigated all these possible pathways on Cu–N 4 and Cu–N 3 SACs. On Cu–N 4 , DFT calculations imply that the first H prefers to bond with C atom of CO 2 to form * HCOO, instead of forming the * HOCO intermediate (the free energy for * HOCO formation is higher than that for * HCOO formation by 0.30 eV at the experimental temperature). * HCOO intermediate then undergoes hydrogenation to form * HCOOH and * H 2 COOH. The formation of * H 2 CO is energetically allowed through the cleavage of C − O bond in * H 2 COOH with the free energy decrease by 0.36 eV (Fig. 4c ). In contrast, DFT calculations indicate that the formation of * HCOO and * HOCO completely occurs on Cu–N 3 SAC, and the free energies for * HCOO and * HOCO are 0.59 and 0.63 eV, respectively (Fig. 4d ). However, the formation of * H 2 COOH via * HCOOH hydrogenation is not allowed by giving a high free energy barrier of 0.75 eV. Consequently, * HOCO is converted into CO via the RWGS pathway. On the other hand, the adsorption energy of CO on Cu–N 3 SAC is only –0.36 eV, indicating that CO can desorb from the surface of catalyst with a free energy decrease of 0.66 eV (Fig. 4d ). Based on the aforementioned results, we conclude that CO 2 hydrogenation follows the formate pathway to form CH 3 OH on Cu–N 4 SAC (Fig. 4e ) and the RWGS pathway to form CO in Cu–N 3 SAC (Fig. 4f ). In summary, we have synthesized C 3 N 4 supported Cu SAC with a high loading amount of 12 wt.% for low temperature CO 2 hydrogenation. By simply altering the parameters for treatment, the coordination structure of Cu atoms in SAC can be systematically tuned by altering the conditions for treatment (e.g., Cu–N 4 and Cu–N 3 ), which leads to the significant differences in the CO 2 hydrogenation. Mechanism studies suggest that the reaction pathways are significantly related to the coordination structure of Cu atoms. In particular, Cu–N 4 SAC exhibits a CH 3 OH productivity of 4.2 mmol g –1 h –1 at a CH 3 OH selectivity of 95.5% at 150 °C, which has surpassed that of commercial Cu/ZnO/Al 2 O 3 by 3.2 times (1 mmol g –1 h –1 ). Detailed investigations show that CO 2 hydrogenation follows the formate pathway to form CH 3 OH on Cu–N 4 SAC and the RWGS pathway to form CO on Cu–N 3 SAC, respectively. This work not only provides an active and selective SAC for low temperature CO 2 hydrogenation, but also sheds lights on studying the structure - performance relationship of catalyst. Chemicals Copper (II) chloride dihydrate (CuCl 2 .2H 2 O, > 99.9%) and melamine were purchased from Shanghai Chemical Reagent company. All chemical reagents were used without further purification. All aqueous solutions were prepared using deionized water with a resistivity of 18.2 MΩ cm –1 . Synthesis of C 3 N 4 In a typical preparation of C 3 N 4 , 500 mg melamine was heated to 550 °C with a rate of 8 °C min –1 in a tube furnace under 5% H 2 /Ar atmosphere for 4 h. After cooling to room temperature, the products were grinded and collected. Synthesis of Cu–N 4 SAC In a typical synthesis of Cu–N 4 SAC, 500 mg melamine, 200 mg CuCl 2 , 5 mL ethanol and 5 mL water were added into a 30 mL vial. The mixture was stirred for 24 h and then centrifuged. The obtained sample was dried in a vacuum oven at 60 °C for 24 h and was thoroughly grinded. Finally, the sample was heated to 550 °C at 8 °C min –1 and maintained at the temperature for 4 h in H 2 /Ar flow (5 vol.% H 2 in Ar). Afterwards, the sample was collected after cooling to room temperature. Synthesis of Cu–N 3 SAC For the synthesis of Cu–N 3 SAC, 100 mg C 3 N 4 and 23 mg CuCl 2 were added into 20 mL ethanol under moderate stirring for 12 h at 80 °C. After that, the product was centrifuged and washed with distilled water and ethanol for three times, followed by drying in vacuum at 70 °C for 24 h. Finally, the sample was heated at 500 °C for 2 h in Ar flow to obtain Cu–N 3 SAC. Synthesis of Cu NPs/C 3 N 4 For the synthesis of Cu NPs/C 3 N 4 , the parameters were same with those of C 3 N 4 supported Cu SACs, except for the final treatment in 0.5 M NaBH 4 for 30 min at room temperature. Characterizations X-ray diffraction (XRD) measurement was conducted on an X’Pert-Pro X-ray powder diffractometer equipped with a Cu radiation source ( λ = 0.15406 nm). High resolution transmission electron microscopy and elemental line scans were performed on a JEOL-2100F transmission electron microscope at an acceleration voltage of 200 kV. High - angle annular dark-field STEM energy-dispersive X-ray spectroscopy (HAADF-STEM-EDS) were conducted on a JEOL GrandARM300F scanning transmission electron microscope with double Cs correctors at an acceleration voltage of 300 kV. Raman spectra were recorded on a HORIBA HR800 instrument. AFM was collected on a Bruker Dimension. Attenuated total reflectance infrared (ATR-IR) spectra were recorded on a Bruker Vertex 70 spectrometer in the spectral range of 4000–400 cm –1 . All the XPS spectra of the Cu NPs were collected by XPS (Thermo Scientific, ESCALAB 250 XI). The concentrations of all the catalysts were determined by the inductively coupled plasma-atomic emission spectroscopy (ICP-AES) (710-ES, Varian). The surface properties like Brunauer–Emmett–Teller surface area, Barrett-Joyner-Halenda (BJH) porosity, pore volume of materials was examined by N 2 adsorption-desorption isotherms at 77 K by using Autosorb Quantachrome 1MP instrument. The in situ Fourier transform infrared (FTIR) spectra of CO adsorption were measured by a Nicolet 6700 equipped with the liquid nitrogen cooled mercury-cadmium-telluride detector (MCT). Quick-scanning X-ray absorption spectroscopy beamline using bending magnet at Taiwan Photon Source (TPS). Catalytic tests The CO 2 hydrogenation was performed in a 60 mL stainless-steel autoclave. The commercial Cu-ZnO/Al 2 O 3 was used as a reference, which was pre-treated in 10%H 2 /Ar at 250 °C for 4 h. After the additions of 10 mL H 2 O and 10 mg catalysts into a Teflon inlet, the autoclave was pressurized with CO 2 (0.8 MPa) and H 2 (2.4 MPa). The reaction was performed at 150 °C with moderate magnetic stirring for 3 h. After completion of the reaction, the gaseous mixture was analyzed using a gas chromatograph (Shiweipx GC-7806) equipped with a GDX-502 column connected to a thermal conductivity detector. The liquid mixture was collected by centrifugation at 14000 × g for 3 min. 10 μL isopropanol was introduced into 1 mL reaction mixture as an internal standard. The liquid mixture was analysed using a gas chromatograph (Persee G5) equipped with a KB-5 column connected to a flame ionization detector. The tests were repeated three times for each catalyst. Theoretical methods DFT calculations were performed by using the Perdew–Burke–Ernzerhof (PBE) functional [37] , [38] within the generalized gradient approximation implemented in Vienna Ab Initio Simulation Package [39] , [40] . The projector-augmented wave method [41] , [42] was applied to describe the electron–ion interactions, and the D3 Grimme’s method was employed to correct van der Waals interaction [43] . We used a plane-wave cutoff energy of 520 eV and the Gaussian smearing with a width of 0.05 eV. Periodic boundary conditions were applied, and more than 15 Å of vacuum space was used to avoid the interaction of the adjacent images. A Γ-centered (3, 3, 1) k -point grid was adopted to sample the Brillouin zone of a 2 × 2 buckled C 3 N 4 supercell with the lattice constant of 6.94 Å. All the structures were fully relaxed until the force components were < 0.02 eV Å –1 . The free energy (G) for each species is expressed as Eq. ( 1 ): 
    G = E_DFT + E_ZPE - TS
 (1) where E DFT , E ZPE , S, and T represents electronic energy, zero-point energy, entropy and temperature (423 K), respectively. The ideal gas approximation and the harmonic approximation were used for H 2 O, H 2 , CO 2 , CO and CH 3 OH molecules, and all atomic nuclear motions for adsorbates were considered as harmonic oscillators. 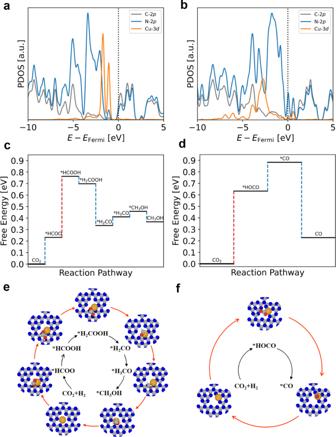Fig. 4: Theoretical calculations and possible reaction paths for CO2hydrogenation. Projected density of states for (a) Cu–N4and (c) Cu–N3SACs, and the Fermi level is indicated by the dashed line. Energy profiles for (b) CO2hydrogenation via formate pathway over Cu–N4SAC and (d) CO2hydrogenation via RWGS pathway over Cu–N3SAC. Reaction pathways and corresponding atomic configurations for CO2hydrogenation to (e) CH3OH and (f) CO. The temperature is set as 423 K. The yellow, blue, gray, red and white balls in (e) and (f) represent as Cu, N, C, O, and H atoms, respectively. The relevant contributions to G were listed in Supplementary Table 4 . A series of gas-phase thermochemical reaction enthalpies (Supplementary Table 5 ) were tested to correct the DFT energies of CO 2 and CO due to the inaccuracy of the PBE functional to describe those molecules [44] . The correction energies of +0.11 and −0.34 eV were applied for CO 2 and CO, respectively. XANES simulations. Cu K-edge XANES spectra were simulated on FDMNES [45] based on the cell structure of Cu–N 4 (Supplementary Fig. 24 ) and Cu–N 3 models (Supplementary Fig. 25 ) used for DFT calculations. Cu reference (ICSD no. 64699) was used for calibrating energy. Hubbard energy of 5 eV was used for all the Cu K-edge simulations [46] , and the Green function employing Muffin-tin potential was applied for the XANES calculations with Athena 0.9.26 [47] . Reporting summary Further information on research design is available in the Nature Research Reporting Summary linked to this article.